Reactivation of a somatic errantivirus and germline invasion inDrosophilaovaries Most Drosophila transposable elements are LTR retrotransposons, some of which belong to the genus Errantivirus and share structural and functional characteristics with vertebrate endogenous retroviruses. Like endogenous retroviruses, it is unclear whether errantiviruses retain some infectivity and transposition capacity. We created conditions where control of the Drosophila ZAM errantivirus through the piRNA pathway was abolished leading to its de novo reactivation in somatic gonadal cells. After reactivation, ZAM invaded the oocytes and severe fertility defects were observed. While ZAM expression persists in the somatic gonadal cells, the germline then set up its own adaptive genomic immune response by producing piRNAs against the constantly invading errantivirus, restricting invasion. Our results suggest that although errantiviruses are continuously repressed by the piRNA pathway, they may retain their ability to infect the germline and transpose, thus allowing them to efficiently invade the germline if they are expressed. Long Terminal Repeat (LTR)-retroelements are a class of transposable elements (TEs) that inhabit nearly all eukaryotic genomes. The genome of Drosophila is largely occupied by a group of insect endogenous LTR-retroelements called errantiviruses, which belong to the Metaviridae family. Errantiviruses share structural and functional characteristics with endogenous retroviruses (ERVs), which are vertebrate LTR-retroelements. Most errantiviruses encode 3 open reading frames (ORFs) whose functions are analogous to that of the Gag, Pol and Env proteins of ERVs or retroviruses. ERVs derive from exogenous retroviruses that integrated into the host germline genome, became permanent elements and are then vertically transmitted. Therefore, they represent a partial record of previous retroviral infections; in Human, ERV-related sequences occupy 9% of the genome, in mice 12%, in rat 10.2%, in microbats 5.3%, in marmosets 7.5% ( http://repeatmasker.org/genomicDatasets/RMGenomicDatasets.html ). Following integration, ERVs are then capable of replicating themselves and integrating at new genomic loci. Each new ERV copy evolves independently and can be at the origin of the emergence of a new TE family. In mice, IAPE and IAP ERVs illustrate the evolutionary history of ERVs [1] . IAPEs are retroviruses capable of infecting other cells after an extracellular passage, whereas highly-repeated IAPs, derived from IAPEs by losing the envelope gene ( env ), are strictly intracellular. Notably, the majority of ERVs are incapable of producing infectious viral particles in vivo. However, insect errantiviruses are not thought to have infectious retroviruses as ancestors and have rather gained potential infectivity independently through the acquisition of a Baculovirus env gene [2] . It is crucial to note that TEs can only be maintained in a species if they are able to transpose into the germline genome. If they do not, they will accumulate mutations until there are no functional copies left, and the TE family dies out. However, some TEs, including ERVs and errantiviruses, gained cell and developmental stage specific expression [3] , [4] , [5] , [6] , [7] . For instance, in the Drosophila melanogaster genome, ZAM, Idefix or Gypsy errantiviruses are expressed exclusively in the somatic follicle cells of the ovaries, with somatic transcription factors controlling their expression [8] , [9] , [10] , [11] , [12] , [13] , [14] , [15] . The Drosophila melanogaster ovary is comprised of about 16 ovarioles, each of which contains a succession of follicles composed of germ cells surrounded by somatic follicle cells [16] . To reach the germline genome, these errantiviruses must then cross the so-called Weismann barrier separating somatic and germ cells. Gypsy and ZAM virus-like particles have been observed in somatic follicle cells. They likely contain the genomic RNA and the expression of the envelope protein could mediate an infection process [8] , [17] . However, the Gypsy envelope is not involved in the soma-to-germline transfer [15] . Instead, it has been proposed that not only Gypsy but also ZAM hijack the host vitellogenic pathway to target the oocyte [11] , [18] . Although the presence of TEs in the genome has been shown to provide some evolutionary benefits (reviewed in [19] ), unregulated TE expression and transposition represent a threat to genome integrity and host fitness. In metazoan gonads, TE expression and mobilization is restrained by PIWI-interacting RNAs (piRNAs) (reviewed in [20] , [21] ). piRNAs originate from specific source loci, the piRNA clusters [22] . In Drosophila gonads, the piRNA clusters expressed in the germline are particularly numerous and diverse, while there is only one major piRNA cluster expressed in gonadal somatic cells, that is flamenco ( flam ) [23] , [24] , [25] , [26] , [27] . Research has primarily concentrated on how piRNAs silence TEs that are expressed in the cells where the corresponding piRNAs are produced. The role of piRNAs in the silencing of a TE that is activated in a cell type different from the one where the silencing mechanism must take place remains unclear. Consequently, whether these TEs can escape the robust epigenetic control mediated by piRNAs when arriving in the germline and how they are tamed by the host over time remained to be puzzled out. The ZAM errantivirus was discovered through its uncontrolled activity in an unstable line, RevI-H2, about 30 years ago [28] , [29] . ZAM has 3 intact ORFs Gag, Pol and Env [28] . In the RevI-H2 Drosophila line bearing a large deletion in the flamenco piRNA cluster, ZAM had become active and is specifically expressed in gonadal somatic cells [8] , [25] . Moreover, ZAM inserted into multiple new loci in the RevI-H2 line, including a germline-specific piRNA cluster, resulting in unexpected production of germline piRNAs that map to ZAM [28] , [29] , [30] . The biological role of these germline ZAM -mapping piRNAs remained unexplored. Since these studies, ZAM has emerged as a key model for studying host-TE interactions and the relationship between somatic cells and the germline during TE invasion. By analyzing different conditions of ZAM reactivation, we aimed here to study what happens when an errantivirus is reactivated de novo and how the host responds. Specifically, we sought to elucidate whether piRNAs produced in the germline counteract TE invasion from the somatic cells or whether TE transcripts are protected from degradation by virus-like particles when arriving in the germline. We show that in the RevI-H2 line, ZAM expression persists in the follicle cells but ZAM does not invade the germline, while ZAM copies with invasive capacities have been maintained in the genome. To recreate the initial unstable condition, we de novo reactivated ZAM in the ovarian follicle cells, either by soma-specific knock-down of the piRNA pathway, or by deleting a ZAM copy in the somatic flamenco piRNA cluster, while keeping the piRNA pathway fully functional. De novo ZAM reactivation in the follicle cells led to a massive ZAM invasion deep into the adjacent oocyte and its ooplasm. We demonstrate that this invasion could be impeded by the expression of de novo ZAM -targeting piRNAs produced in the germ cells themselves, demonstrating that these piRNAs are functional against the native ZAM . These results show that by being expressed exclusively in somatic cells, errantiviruses may evade the highly efficient control of the germline piRNA pathway and remain active for long periods of time (in the case of the RevI-H2 line, at least 30 years). The challenged germ cells then mount an adaptive genomic immune response to tackle the permanent invasion. In an ancient flamenco mutant line, ZAM is still expressed, but the line is nevertheless stable To investigate the history of ZAM transposition dynamics, we monitored ZAM copies in the RevI-H2i2 line, an isogenic line that was recently derived from the parental flam mutant RevI-H2 line that has more than 25 years of laboratory history. It had previously been reported that the RevI-H2 line was unstable and that ZAM actively transposed in this line [29] . The ZAM instability in RevI-H2 had been linked to a deletion of a large part of the flam piRNA cluster. This deletion spanned over more than 120 kb and comprised many different TE relics, including more or less recent copies, and all ZAM -related copies of the flam locus [25] , [26] . In the RevI-H2i2 genome, Oxford Nanopore Technology (ONT) genome sequencing revealed 18 ZAM copies (Fig. 1a and Supplementary Data 1 for coordinates). Only one of these ZAM copies was also present in the reference genome ( http://flybase.org ). The other 17 new insertions were very similar to the ZAM reference element identified in the initial RevI-H2 line [28] and we could clearly localize 14 of the 17 new ZAM insertions. Interestingly, ONT long-read sequencing, allowed identifying different ZAM variants. Specifically, six were full-length ZAM elements (ZAM-fl), one, named ZAM-v1, harbored a deleted 5’-UTR (5’ untranslated region), two, named ZAM-v3, had a 303 bp deletion within the 5’-UTR, four had large internal deletions in the coding regions, and four were full-length insertions with a deletion at the C-terminal end of the pol gene of positions 5494 to 6120 in the ZAM internal sequence [28] (Repbase ZAM_I, https://www.girinst.org/repbase/ [31] ). This deleted part of the pol gene does not correspond to any known protein domain, and the fact that there are five identical copies of this ZAM at different locations in the RevI-H2i2 genome indicates that this ZAM variant, which we named ZAM-v2, is competent for transposition. The full-length ZAM , ZAM-v1 and ZAM-v3 copies all potentially encode Gag, Pol and Env proteins (Fig. 1a ). Fig. 1: ZAM is expressed in follicle cells in the RevI-H2i2 isogenic line but the line is stable. a ZAM elements in the RevI-H2i2 genome. Each triangle represents a ZAM insertion. The different ZAM variants are presented in the illustration on the right. The positions refer to ZAM internal sequences (ZAM_I in RepBase). Blue: full-length ZAM elements (ZAM-fl); violet: ZAM variants ZAM-v1 with deleted 5’-UTR; orange: ZAM variants ZAM-v2, in which positions 5494-6120 are deleted; yellow: ZAM variants ZAM-v3 with a 303 bp deletion in the 5’-UTR; green: ZAM with internal deletions other than ZAM variants above; gray: full-length ZAM copy also present in the reference Release 6 genome ( http://flybase.org ). The dotted box indicates four ZAM copies on the X chromosome inserted in referenced germline piRNA clusters (Cluster 9 and 13 ). No ZAM insertion was found in chromosome 4 (1.35 Mb, see Supplementary Data 1 ). For coordinates and details see Supplementary Data 1 . b Projection of confocal images of ovarioles, germarium, and stage 10 follicles showing ZAM expression by smRNA FISH (in red) in RevI-H2i2 ovaries. DNA was stained with DAPI (white). The experiment was independently repeated at least 10 times, with similar results obtained each time. c Fold-change in the steady-state ZAM , Gypsy and Burdock RNA levels for RevI-H2i2 ovaries compared with w 1118 ovaries (control), quantified by RT-qPCR (primer sequences in Supplementary Data 5 ). n = 3 biological independent samples and two reverse transcription experiments have been performed for each replicate, resulting in a total of six data points per genotype. All data points are shown as dot plots. ** p value = 0,0087; ns, not significant ( p value > 0.05) (Mann-Whitney two-sided test). Data are presented as mean values and the error bars indicate the standard deviation from the mean values. d Confocal sections of stage 10 egg chambers of RevI-H2i2 and w 1118 control line showing ZAM -encoded Gag (green) and Env (red) proteins. DNA was stained with DAPI (white). The experiment was independently repeated at least 5 times, with similar results obtained each time. e Morphology of control and RevI-H2i2 ovaries. f Box plot displaying the number of eggs laid per fly per day by control and RevI-H2i2 females. Each dot represents an individual female. The experiment was repeated twice for each condition to reach n = 60 control females, n = 63 RevI-H2i2 females. In the box plots, the midline corresponds to the median value; the lower and upper hinges correspond to the first and third quartiles; and the whiskers span the minimum and maximum values, excluding outliers. ns, not significant ( p value > 0.05) (Mann-Whitney two-sided test). Full size image In the initial RevI-H2 line, a ZAM insertion was found in the germline piRNA cluster 9 , which is close to the X chromosome centromere [30] . Here, in the RevI-H2i2 line, thanks to long-read sequencing, we could identify ZAM insertions in repeated sequences, such as piRNA clusters, more accurately. We now identified three ZAM insertions in piRNA cluster 9 (one ZAM-fl and two ZAM-v2), and also a ZAM-fl insertion, which is localized in either piRNA cluster 13 or cluster 56 (uncertainty is due to flanking repeats, piRNA clusters as in [32] ) (Fig. 1a ). We reanalyzed the Illumina sequencing data of the initial RevI-H2 line and found evidence that all these ZAM insertions in piRNA cluster 9 and 13 or 56 were already present ten years ago, and that at least 14 of the ZAM insertions in the RevI-H2i2 line were already present in the parental RevI-H2 line. This result indicates that the genomic ZAM profile is the same as ten years ago and suggests that no new ZAM insertions occurred since then in the germline. Strikingly, no new ZAM insertion was detected in the flam piRNA cluster. Thus, in the RevI-H2i2 line, no ZAM piRNA can be produced from flam , the major somatic piRNA source locus. Interestingly, single-molecule RNA fluorescence in situ hybridization (smRNA FISH) revealed the presence of ZAM RNA in RevI-H2i2 follicle cells, demonstrating that ZAM is not silenced in these somatic cells and that transcriptionally active copies of ZAM are still present in the genome. ZAM transcripts were produced in follicle cells, starting very early during oogenesis in the germarium. Then, after stage 8, ZAM transcripts accumulated in a patch of follicle cells located at the posterior side of the follicles. We did not detect any ZAM staining in germ cells (nurse cells or oocytes) (Fig. 1b ). 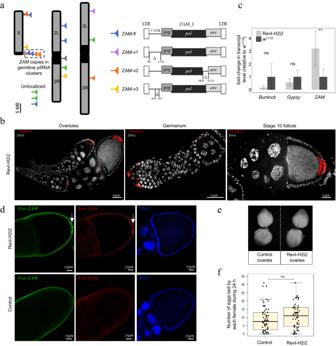Fig. 1:ZAMis expressed in follicle cells in the RevI-H2i2 isogenic line but the line is stable. aZAMelements in the RevI-H2i2 genome. Each triangle represents aZAMinsertion. The differentZAMvariants are presented in the illustration on the right. The positions refer toZAMinternal sequences (ZAM_I in RepBase). Blue: full-lengthZAMelements (ZAM-fl); violet:ZAMvariants ZAM-v1 with deleted 5’-UTR; orange:ZAMvariants ZAM-v2, in which positions 5494-6120 are deleted; yellow: ZAM variants ZAM-v3 with a 303 bp deletion in the 5’-UTR; green:ZAMwith internal deletions other thanZAMvariants above; gray: full-lengthZAMcopy also present in the reference Release 6 genome (http://flybase.org). The dotted box indicates fourZAMcopies on the X chromosome inserted in referenced germline piRNA clusters (Cluster9and13). NoZAMinsertion was found in chromosome 4 (1.35 Mb, see Supplementary Data1). For coordinates and details see Supplementary Data1.bProjection of confocal images of ovarioles, germarium, and stage 10 follicles showingZAMexpression by smRNA FISH (in red) in RevI-H2i2 ovaries. DNA was stained with DAPI (white). The experiment was independently repeated at least 10 times, with similar results obtained each time.cFold-change in the steady-stateZAM,GypsyandBurdockRNA levels for RevI-H2i2 ovaries compared withw1118ovaries (control), quantified by RT-qPCR (primer sequences in Supplementary Data5).n= 3 biological independent samples and two reverse transcription experiments have been performed for each replicate, resulting in a total of six data points per genotype. All data points are shown as dot plots. **pvalue = 0,0087; ns, not significant (pvalue > 0.05) (Mann-Whitney two-sided test). Data are presented as mean values and the error bars indicate the standard deviation from the mean values.dConfocal sections of stage 10 egg chambers of RevI-H2i2 andw1118control line showingZAM-encoded Gag (green) and Env (red) proteins. DNA was stained with DAPI (white). The experiment was independently repeated at least 5 times, with similar results obtained each time.eMorphology of control and RevI-H2i2 ovaries.fBox plot displaying the number of eggs laid per fly per day by control and RevI-H2i2 females. Each dot represents an individual female. The experiment was repeated twice for each condition to reachn= 60 control females,n= 63 RevI-H2i2 females. In the box plots, the midline corresponds to the median value; the lower and upper hinges correspond to the first and third quartiles; and the whiskers span the minimum and maximum values, excluding outliers. ns, not significant (pvalue > 0.05) (Mann-Whitney two-sided test). RNase A treatment led to complete loss of ZAM staining in the follicle cells (Supplementary Figure 1a ). We did not detect any ZAM RNA in the Iso1A, w 1118 and w IR6 control ovaries (Supplementary Figure 1b ). Using RT-qPCR, we confirmed that ZAM was expressed in the RevI-H2i2 ovaries. Conversely, other TEs such as the soma-specific Gypsy and the germline-specific Burdock , were not upregulated (Fig. 1c ). Interestingly, we observed that, besides the full-length ZAM, at least ZAM variants ZAM-v2 and ZAM-v3 are expressed in RevI-H2i2 ovaries (Supplementary Figure 1c, d ). ZAM is an errantivirus that encodes Gag, Pol and Env proteins. Using immunostaining, we were able to detect ZAM Gag and Env proteins that accumulated in the posterior follicle cells in late-stage follicles ( > stage 9) (Fig. 1d ). All these results showed that ZAM transcripts and proteins are still expressed in the RevI-H2i2 line. Although ZAM was expressed in follicle cells, the RevI-H2i2 line was fertile. Indeed, the ovary morphology and the number of eggs laid were comparable in RevI-H2i2 and control females (Fig. 1e, f ). Altogether, these results indicate that no silencing mechanism had been set up to repress the ZAM errantivirus in follicle cells, suggesting that ZAM expression has no major deleterious effect in the RevI-H2i2 line and that there is no selective pressure to specifically repress ZAM in the follicles cells. These findings suggest that RevI-H2i2 is a stable line although ZAM is actively expressed in follicle cells. Germline ZAM- targeting piRNAs constrain ZAM invasion from adjacent somatic cells Transposition of ZAM in the initial RevI-H2 line had occurred in the germline, as attested by the transmission of ZAM insertions to the offspring, despite the fact that ZAM is specifically and exclusively expressed in the somatic follicle cells. This confirms that the ZAM errantivirus, when expressed in follicle cells, transits to the germline to integrate into the germ cell genome. However, we showed that ZAM insertions are stabilized in the RevI-H2i2 line. The RevI-H2i2 flies produce high amounts of sense and antisense ZAM -derived piRNAs with a ping-pong signature, revealed by an over-representation of 10-nucleotide 5’-overlaps between sense and antisense ZAM -derived piRNAs (Fig. 2a ), while there was no ping-pong signature for ZAM in diverse control lines [14] , [30] . Ping-pong amplification of piRNAs can only occur in the germline in Drosophila (reviewed in [33] ). Thus, these ZAM piRNAs observed in RevI-H2i2 are derived from the germline. Importantly, our previous research has demonstrated that the X chromosome of the RevI-H2 line, which contains the ZAM copies inserted in germline piRNA clusters, is both necessary and sufficient to produce ZAM -regulating piRNAs [30] . 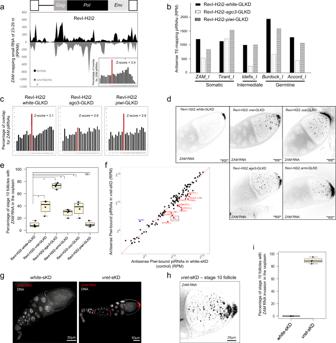Fig. 2: GermlineZAMpiRNAs produced in RevI-H2i2 germ cells counteractZAMinvasion. aDensity plot ofZAM-mapping regulatory piRNAs along theZAMsequence in RevI-H2i2 ovaries (up to 3 mismatches). In the lower right corner is the histogram showing the percentage of 5’-overlaps between sense and antisenseZAM-derived piRNAs (23–29 nt) in RevI-H2i2 ovaries. The proportion of 10nt 5’-overlaps is in red and the corresponding Z-score is indicated.bAntisense piRNAs mapping to TE internal sequences (0-3 mismatches) in the RevI-H2i2 line uponwhite-(control),ago3-, orpiwi-GLKD. Normalized per million of genome-mapping piRNAs.cHistogram showing the percentage of 5’-overlaps between sense and antisenseZAM-mapping piRNAs (up to 3 mismatches) inwhite-, ago3-, orpiwi-GLKD RevI-H2i2 ovaries. The percentage of 10nt overlaps is in red and the corresponding Z-score is indicated.dColor-inverted confocal images of stage 10 egg chambers showingZAMsmRNA FISH signal in ovaries of the indicated genotypes.eBar plot showing the percentage of stage 10 follicles withZAMRNA detected in the ooplasm by smRNA FISH of RevI-H2i2 ovaries with the indicated GLKD. This experiment was done four times resulting in a total number ofn= 172 for RevI-H2i2white-GLKD,n= 105 for RevI-H2i2vret-GLKD,n= 160 RevI-H2i2ago3-GLKD follicles,n= 168 for RevI-H2i2armi-GLKD,n= 172 for RevI-H2i2 white GLKD,n= 109 for RevI-H2i2zuc-GLKD,n= 97 for RevI-H2i2piwi-GLKD independent stage 10 follicles. In the box plots, the midline corresponds to the median value; the lower and upper hinges correspond to the first and third quartiles; and the whiskers span the minimum and maximum values, excluding outliers. *:pvalue = 0.02857; ns, not significant (pvalue = 0,8857) (Mann-Whitney, two-sided test).fScatter plot showing the normalized counts of antisense Piwi-bound piRNAs mapping to individual internal TEs sequences in control ovaries (white-sKD) andvret-sKD ovaries. Antisense piRNA counts, mapped allowing up to 3 mismatches, were normalized per million of genome-mapping piRNAs (RPM, here in logarithmic scale). TEs in red have avret-sKD/white-sKD ratio <0.3.ZAMis boxed black.gConfocal images of ovarioles showingZAMsmRNA FISH signal (in red) inwhite- (control) and vret-sKD ovaries. DNA was stained with DAPI (white).hColor-inverted confocal projection of stage 10 egg chamber showingZAM smRNA FISH signal invret-sKD ovaries.iBar plot showing the percentage of stage 10 follicles withZAMRNA invasion of the ooplasm, assessed byZAMsmRNA FISH, ofwhite- (control) andvret-sKD ovaries. This experiment was done 4 times resulting in a total number ofn= 116white-sKD andn= 98vret-sKD independent stage 10 follicles. In the box plots, the midline corresponds to the median value; the lower and upper hinges correspond to the first and third quartiles; and the whiskers span the minimum and maximum values, excluding outliers. Additionally, in both RevI-H2 [30] and RevI-H2i2 background, a ZAM sensor transgene is silenced in the germ cells (Supplementary Figure 2a ). We therefore hypothesized that piRNAs produced in germ cells can thwart ZAM invasion from somatic cells to the germline and thus protect the germline from new ZAM transposition. However, piRNAs are known to silence TEs in the cells where they are produced and some TEs, such as ZAM , are not expressed directly in germ cells but arrive from surrounding somatic cells. Moreover, ZAM RNA may transit in an encapsulated form and the capacity of piRNAs to target encapsulated RNAs remains unknown. Fig. 2: Germline ZAM piRNAs produced in RevI-H2i2 germ cells counteract ZAM invasion. a Density plot of ZAM -mapping regulatory piRNAs along the ZAM sequence in RevI-H2i2 ovaries (up to 3 mismatches). In the lower right corner is the histogram showing the percentage of 5’-overlaps between sense and antisense ZAM -derived piRNAs (23–29 nt) in RevI-H2i2 ovaries. The proportion of 10nt 5’-overlaps is in red and the corresponding Z-score is indicated. b Antisense piRNAs mapping to TE internal sequences (0-3 mismatches) in the RevI-H2i2 line upon white- (control), ago3- , or piwi -GLKD. Normalized per million of genome-mapping piRNAs. c Histogram showing the percentage of 5’-overlaps between sense and antisense ZAM -mapping piRNAs (up to 3 mismatches) in white-, ago3- , or piwi- GLKD RevI-H2i2 ovaries. The percentage of 10nt overlaps is in red and the corresponding Z-score is indicated. d Color-inverted confocal images of stage 10 egg chambers showing ZAM smRNA FISH signal in ovaries of the indicated genotypes. e Bar plot showing the percentage of stage 10 follicles with ZAM RNA detected in the ooplasm by smRNA FISH of RevI-H2i2 ovaries with the indicated GLKD. This experiment was done four times resulting in a total number of n = 172 for RevI-H2i2 white -GLKD, n = 105 for RevI-H2i2 vret -GLKD, n = 160 RevI-H2i2 ago3 -GLKD follicles, n = 168 for RevI-H2i2 armi -GLKD, n = 172 for RevI-H2i2 white GLKD, n = 109 for RevI-H2i2 zuc -GLKD, n = 97 for RevI-H2i2 piwi -GLKD independent stage 10 follicles. In the box plots, the midline corresponds to the median value; the lower and upper hinges correspond to the first and third quartiles; and the whiskers span the minimum and maximum values, excluding outliers. *: p value = 0.02857; ns, not significant ( p value = 0,8857) (Mann-Whitney, two-sided test). f Scatter plot showing the normalized counts of antisense Piwi-bound piRNAs mapping to individual internal TEs sequences in control ovaries ( white -sKD) and vret -sKD ovaries. Antisense piRNA counts, mapped allowing up to 3 mismatches, were normalized per million of genome-mapping piRNAs (RPM, here in logarithmic scale). TEs in red have a vret -sKD/ white -sKD ratio <0.3. ZAM is boxed black. g Confocal images of ovarioles showing ZAM smRNA FISH signal (in red) in white - (control) and v ret -sKD ovaries. DNA was stained with DAPI (white). h Color-inverted confocal projection of stage 10 egg chamber showing ZAM sm RNA FISH signal in vret -sKD ovaries. i Bar plot showing the percentage of stage 10 follicles with ZAM RNA invasion of the ooplasm, assessed by ZAM smRNA FISH, of white - (control) and vret -sKD ovaries. This experiment was done 4 times resulting in a total number of n = 116 white -sKD and n = 98 vret -sKD independent stage 10 follicles. In the box plots, the midline corresponds to the median value; the lower and upper hinges correspond to the first and third quartiles; and the whiskers span the minimum and maximum values, excluding outliers. Full size image To test whether germline ZAM -derived piRNAs were efficient to counteract an invasion coming from surrounding somatic cells, we abolished the piRNA pathway in the germ cells by germline-specific knock-down (GLKD) of piRNA pathway components, in a RevI-H2i2 genetic background producing ZAM piRNAs in the germline. It is important to note that, during the genetic crosses performed, only the X chromosome of the RevI-H2i2 was tracked to ensure that the ZAM insertions in the germline piRNA clusters were maintained ( Drosophila lines for knock-down are listed in Supplementary Data 2 , crossing schemes presented in Supplementary Figure 6 ). We observed that the germline knock-down of proteins of the piRNA pathway, Zucchini (Zuc), Argonaute 3 (Ago3) and Piwi, led to a decrease in the production of ZAM- targeting piRNAs, i.e. piRNAs that are complementary and thus antisense to ZAM (Fig. 2b , Supplementary Figure 2b ). The decrease in antisense piRNAs was comparable to that observed for germline TEs (i.e., Burdock and Accord ) or intermediate TEs (i.e., Idefix ), while the level of piRNA of somatic TEs, such as Tirant , was not affected. Furthermore, in ago3 -GLKD ovaries, the ping-pong signature for ZAM was abolished, as for many other germline-specific TEs, while it was maintained in piwi- GLKD ovaries, for instance (Fig. 2c , Supplementary Figure 2c ). We then analyzed the subcellular localization of ZAM RNAs by smRNA FISH in the RevI-H2i2 white -GLKD control line in which ZAM -derived piRNAs are produced in the germline. ZAM RNA staining was restricted to follicle cells, only a minor ZAM RNA signal was detected in the posterior pole of approximately 10% of stage 10 oocytes (Fig. 2d, e ). However, when the piRNA pathway was abolished in RevI-H2i2 germ cells through vreteno (vret) , zuc, ago3 or armitage (armi) GLKD, ZAM RNA was no longer restricted to follicle cells, a high signal was also detected in oocytes. ZAM RNA spread throughout the ooplasm, but was clearly enriched at the posterior pole of the oocyte, adjacent to the ZAM -expressing follicle cells, supporting the fact that ZAM RNA originated from follicle cells (Fig. 2d ). Actually, 30-70% of stage 10 follicles showed a strong ZAM RNA signal in oocytes (Fig. 2e ). The strongest invasion phenotype was observed for the RevI-H2i2 ago3 -GLKD condition where we found a decrease in the production of ZAM -derived piRNAs and the loss of the ping-pong signature (Fig. 2b ). In this condition, ZAM RNA accumulation in the ooplasm was correlated with a strong increase of ZAM RNA in total ovaries (RT-qPCR data) (Supplementary Figure 2d ). These results showed that when the piRNA pathway is affected in the germline , ZAM RNAs transit from the somatic follicle cells, where they are produced, to the oocyte. Altogether, our data strongly suggest that ZAM piRNAs produced by the germline piRNA pathway trigger post-transcriptional silencing of ZAM RNAs arriving from follicle cells. We confirmed this finding using a line where no ZAM -derived piRNA is produced in the germline ( w 1118 genetic background) and in which we knocked down the piRNA pathway in the follicle cells by somatic knock-down (sKD) of armi , vret , piwi or yb . The amount of antisense piRNAs that target soma-specific TEs, including ZAM , was strongly decreased (Fig. 2f , Supplementary Figure 2e, f ). RT-qPCR analysis showed that ZAM and another soma-specific TE, Gypsy , were derepressed, but not the germline-specific Burdock (Supplementary Figure 2g ). Importantly, smRNA FISH results revealed that ZAM RNAs were not restricted to the posterior follicle cells. Like in ovaries harboring GLKD of the piRNA pathway in RevI-H2i2 background, ZAM RNAs were present in oocytes (Fig. 2g, h , Supplementary Figure 2h ). We detected ZAM RNAs in the ooplasm in 90% of stage 10 follicles (Fig. 2i ). This result confirmed that, when no ZAM piRNA is produced in the germline, ZAM RNAs expressed in the somatic follicle cells transit to the oocyte and then persist in the oocyte. ZAM RNAs transcribed in follicle cells transit to the oocyte and are conveyed to the embryos in the absence of germline ZAM piRNAs Although ZAM is expected to be transcribed only in follicle cells due to its dependence on the Pointed somatic transcription factor [8] , [34] , it was possible that some ZAM copies acquired the capacity to be expressed in the germline over time. Therefore, we wanted to rule out the possibility that ZAM RNAs detected in the RevI-H2i2 oocyte originated from germinal nurse cells. If some ZAM genomic insertions could be expressed in the germline of the RevI-H2i2 line, then germline depletion of Piwi , which is required for the transcriptional gene silencing of TEs, should lead to the transcriptional de-silencing of ZAM . We observed that Piwi-GLKD in the RevI-H2i2 ovaries led to the de-silencing of TEs that are capable of transcribing in the germline, such as Burdock . However, we did not observe any changes in either the ZAM RNA level or localization (Fig. 3a, b ). Moreover, the depletion of Ago3 induced a substantial accumulation of ZAM RNA solely in the ooplasm. In contrast to TEs expressed in the germline (e.g, Burdock ), we never detected ZAM RNA staining in the cytoplasm of the nurse cells at any stage (Fig. 3c ). These results strongly support that ZAM cannot be expressed in the RevI-H2i2 germ cells and that ZAM RNAs detected in oocytes originate from the somatic follicle cells, not nurse cells. Fig. 3: ZAM RNAs transcribed in the follicle cells transit to the oocyte and are deposited in early embryos. a Confocal images of stage 10 follicles in the RevI-H2i2 piwi -GLKD line. Burdock (green) and ZAM (red) mRNAs were detected by smRNA FISH. DNA was stained with DAPI (blue). The experiment was independently repeated at least 5 times, with similar results obtained each time. b Fold-change in the steady-state ZAM , Burdock and Piwi RNA levels for RevI-H2i2 piwi- GLKD ovaries compared with RevI-H2i2 white- GLKD ovaries (control), quantified by RT-qPCR (primer sequences in Supplementary Data 5 ). n = 3 biological independent samples and two technical replicates have been performed for each sample, resulting in a total of six data points per genotype. All data points are shown as dot plots. *: p value = 0,022, **: p value = 0,008; ns, not significant ( p value > 0.05) (Mann-Whitney two-sided test). Data are presented as mean values and the error bars indicate the standard deviation from the mean values. c Confocal images of ovarioles and of an isolate stage 8 egg chamber in the RevI-H2i2 ago3 -GLKD line. Burdock (green) and ZAM (red) mRNAs were detected by smRNA FISH. DNA was stained with DAPI (blue). The experiment was independently repeated at least 5 times, with similar results obtained each time. d Color-inverted confocal images showing ZAM smRNA FISH signal in early embryos collected 0–2 hours after egg laying (AEL). Mothers were from the indicated genotype. The experiment was independently repeated at least 3 times, with similar results obtained each time. e Zoom on the posterior part of a vret -sKD early embryo collected at 0–1 hours AEL showing ZAM RNA accumulation at the posterior pole. The experiment was independently repeated at least 5 times, with similar results obtained each time. f Color-inverted confocal images showing ZAM smRNA FISH signal in embryos laid by vret -sKD females at the indicated developmental stages. The experiment was independently repeated at least 3 times, with similar results obtained each time. Full size image Throughout the animal kingdom, the first embryonic development stages are controlled by transcripts and proteins deposited by the mother during oogenesis [35] . In Drosophila , most of the maternal mRNAs are dumped from nurse cells into the oocyte during oogenesis. Although ZAM transcripts originate from the somatic follicle cells, when we investigated ZAM RNA transmission to the oocyte, we found such transcripts also in early embryos. Indeed, in conditions where ZAM RNA had been detected in oocytes, smRNA FISH experiments revealed a strong accumulation of ZAM RNAs in early embryos, before the zygotic transition, 0-2 hours after egg laying: from a RevI-H2i2 mother with GLKD of the piRNA pathway, and also from a mother without germinal ZAM piRNAs with sKD of the piRNA pathway in follicle cells (Fig. 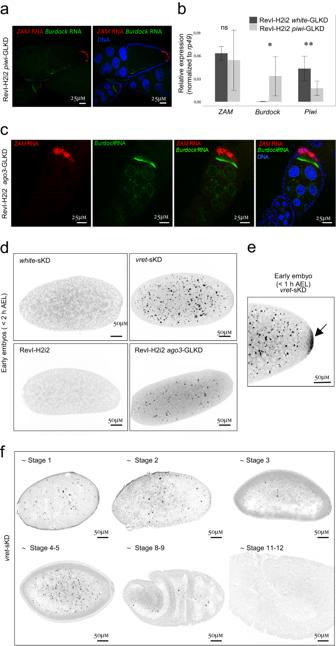Fig. 3:ZAMRNAs transcribed in the follicle cells transit to the oocyte and are deposited in early embryos. aConfocal images of stage 10 follicles in the RevI-H2i2piwi-GLKD line.Burdock(green) andZAM(red) mRNAs were detected by smRNA FISH. DNA was stained with DAPI (blue). The experiment was independently repeated at least 5 times, with similar results obtained each time.bFold-change in the steady-stateZAM,BurdockandPiwiRNA levels for RevI-H2i2piwi-GLKD ovaries compared with RevI-H2i2white-GLKD ovaries (control), quantified by RT-qPCR (primer sequences in Supplementary Data5).n= 3 biological independent samples and two technical replicates have been performed for each sample, resulting in a total of six data points per genotype. All data points are shown as dot plots. *:pvalue = 0,022, **:pvalue = 0,008; ns, not significant (pvalue > 0.05) (Mann-Whitney two-sided test). Data are presented as mean values and the error bars indicate the standard deviation from the mean values.cConfocal images of ovarioles and of an isolate stage 8 egg chamber in the RevI-H2i2ago3-GLKD line.Burdock(green) andZAM(red) mRNAs were detected by smRNA FISH. DNA was stained with DAPI (blue). The experiment was independently repeated at least 5 times, with similar results obtained each time.dColor-inverted confocal images showingZAMsmRNA FISH signal in early embryos collected 0–2 hours after egg laying (AEL). Mothers were from the indicated genotype. The experiment was independently repeated at least 3 times, with similar results obtained each time.eZoom on the posterior part of avret-sKD early embryo collected at 0–1 hours AEL showingZAMRNA accumulation at the posterior pole. The experiment was independently repeated at least 5 times, with similar results obtained each time.fColor-inverted confocal images showingZAMsmRNA FISH signal in embryos laid byvret-sKD females at the indicated developmental stages. The experiment was independently repeated at least 3 times, with similar results obtained each time. 3d , Supplementary Figure 3a ). Furthermore, ZAM RNAs accumulated at the posterior pole of early embryos where future germ cells cellularize (Fig. 3e , Supplementary Figure 3b ). We detected ZAM RNA in high quantity until stage 5 of embryogenesis and few ZAM RNA signal persisting until the cellularization of the blastoderm ( ~ stage 8-9) (Fig. 3f ). In the progeny of the RevI-H2i2 line, we did not detect any ZAM RNA, although ZAM RNAs were produced in follicle cells of RevI-H2i2 ovaries (Fig. 3d ). This confirmed that ZAM invasion of the germline does not occur in this line. These data revealed an efficient post-transcriptional silencing of ZAM RNAs arriving from follicle cells into the oocyte by piRNAs produced in the germline. This mechanism should limit the transposition of the somatic ZAM retrotransposon into the germline genome. De novo ZAM reactivation leads to massive oocyte invasion and may result in severe fertility defects Our results demonstrate that an adaptive response can emerge to counteract the invasion of germ cells by an errantivirus. To go deeper, we sought to assess the direct impact of reactivating an errantivirus de novo, before the establishment of any adaptive response by the germline. To conduct this study, we aimed to specifically reactivate ZAM de novo. The loss of the piRNA pathway in the somatic follicle cells leads to ZAM reactivation, however, many other TEs are also desilenced (Supplementary Figure 2e, g ). Moreover, alteration in the expression of piRNA pathway genes also results in severe developmental defects during oogenesis [36] , [37] , [38] , [39] . Therefore, this model cannot be used to specifically analyze the impact of ZAM reactivation in ovaries. On the other hand, in the RevI-H2 line where ZAM was also reactivated, a large deletion of flamenco occurred during non-targeted mutagenesis and an adaptive response had already been set up in the germline. Thus, we chose to create a condition where a single TE is reactivated de novo and the piRNA pathway is fully functional. Using CRISPR-Cas9, we de novo deleted the longest ZAM copy in the flam piRNA cluster in a line carrying the X chromosome of the Iso1A reference line. As in this line, the flam ZAM copy is at the genomic position X:21,778,810..21,783,994, we used two guides designed to create a deletion spanning over X:21,777,135..21,784,062 (6926 pb). We named the resulting line flamΔZAM . Mapping of genome-unique piRNAs to the flam locus highlighted the complete loss of piRNA production in the targeted region compared with the control Iso1A line (Fig. 4a ). Conversely, the global production of genome-unique piRNAs mapping upstream and downstream of ZAM was not affected. We confirmed that the deletion induced a strong decrease of all piRNAs mapping to the internal regions of the reference ZAM . However, piRNAs targeting the ZAM LTR were still produced (Fig. 4b ). 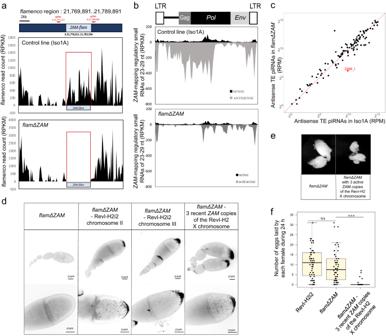Fig. 4:ZAMdeletion from theflamencopiRNA cluster leads toZAMreactivation and oocyte invasion. aDensity plots showing genome-unique piRNAs mapping over 20 kb of theflamencopiRNA cluster (without mismatch) where theZAMinsertion is located (Release 6: X:21,769,891..21,789,891) in the control (Iso1A) andflamΔZAMlines. The position of theflamenco ZAMcopy(ZAM-flam)is indicated. The positions of the sgRNAs used forZAM-flamdeletion by CRISPR-Cas9 are shown in red.bDensity plot ofZAM-mapping regulatory piRNAs along theZAMsequence in control andflamΔZAMovaries (up to 3 mismatches).cScatter plot showing the normalized counts of antisense regulatory piRNAs mapping to individual internal TE sequences in control ovaries (Iso1A) versusflamΔZAMovaries. Antisense piRNA counts, mapped allowing up to 3 mismatches, were normalized per million of genome-mapping piRNAs (RPM, here in logarithmic scale). TEs in red have aflamΔZAM/Iso1A ratio <0.3.dColor-inverted confocal images of ovarioles (upper panels) and stage 10 egg chambers (lower panels) from the indicated genotypes showingZAMsmRNA FISH signal. The experiment was independently repeated at least 5 times, with similar results obtained each time.eOvaries of theflamΔZAMline and of theflamΔZAMline with three recentZAMcopies introduced by genetic crossing and X chromosome recombination with the RevI-H2 line.fBox plot displaying the number of eggs laid per fly per day by RevI-H2i2,flamΔZAM and flamΔZAMfemales with three recentZAMcopies. Each dot represents an individual female.n= 63 for RevI-H2i2,n= 60 forflamΔZAM,n= 60 forflamΔZAMwith three recentZAMcopies. In the box plots, the midline corresponds to the median value; the lower and upper hinges correspond to the first and third quartiles; and the whiskers span the minimum and maximum values, excluding outliers. ***pvalue < 2.2e-16; ns, not significant (pvalue > 0.05) (Mann-Whitney two-sided test). In line with these results, PCR amplification and DNA sequencing of the CRISPR-Cas9 target locus showed that only the internal regions of ZAM had been deleted from the flam piRNA cluster, resulting in the retention of a solo-LTR at the initial ZAM insertion site (Supplementary Figure 4a ). Fig. 4: ZAM deletion from the flamenco piRNA cluster leads to ZAM reactivation and oocyte invasion. a Density plots showing genome-unique piRNAs mapping over 20 kb of the flamenco piRNA cluster (without mismatch) where the ZAM insertion is located (Release 6: X:21,769,891..21,789,891) in the control (Iso1A) and flam Δ ZAM lines. The position of the flamenco ZAM copy (ZAM-flam) is indicated. The positions of the sgRNAs used for ZAM-flam deletion by CRISPR-Cas9 are shown in red. b Density plot of ZAM -mapping regulatory piRNAs along the ZAM sequence in control and flamΔZAM ovaries (up to 3 mismatches). c Scatter plot showing the normalized counts of antisense regulatory piRNAs mapping to individual internal TE sequences in control ovaries (Iso1A) versus flamΔZAM ovaries. Antisense piRNA counts, mapped allowing up to 3 mismatches, were normalized per million of genome-mapping piRNAs (RPM, here in logarithmic scale). TEs in red have a flamΔZAM /Iso1A ratio <0.3. d Color-inverted confocal images of ovarioles (upper panels) and stage 10 egg chambers (lower panels) from the indicated genotypes showing ZAM smRNA FISH signal. The experiment was independently repeated at least 5 times, with similar results obtained each time. e Ovaries of the flamΔZAM line and of the flamΔZAM line with three recent ZAM copies introduced by genetic crossing and X chromosome recombination with the RevI-H2 line. f Box plot displaying the number of eggs laid per fly per day by RevI-H2i2, flamΔZAM and flamΔZAM females with three recent ZAM copies. Each dot represents an individual female. n = 63 for RevI-H2i2, n = 60 for flamΔZAM , n = 60 for flamΔZAM with three recent ZAM copies. In the box plots, the midline corresponds to the median value; the lower and upper hinges correspond to the first and third quartiles; and the whiskers span the minimum and maximum values, excluding outliers. *** p value < 2.2e-16; ns, not significant ( p value > 0.05) (Mann-Whitney two-sided test). Full size image In the flamΔZAM line , only the production of ZAM -derived antisense piRNAs was strongly altered, whereas the production of antisense piRNAs mapping to other TEs was not affected (Fig. 4c ). This shows that the ZAM deletion from flam impairs ZAM -derived piRNA production, but does not affect the global piRNA production in ovaries. In sum, in the flamΔZAM line, the piRNA pathway was functional and almost no piRNAs that could target the internal ZAM sequences were produced. We then analyzed ZAM RNA expression by smRNA FISH in flamΔZAM ovaries. Surprisingly, we did not detect any ZAM expression (Fig. 4d – panel 1). Based on this observation, we hypothesized that either there was no functional ZAM copy in the flamΔZAM line, or that the ZAM solo-LTR retained in flam was sufficient to silence ZAM expression. To check this, we exchanged chromosome II or III of the flamΔZAM line with chromosome II or III of the RevI-H2i2 line that each contains three or two recently transposed potentially functional ZAM copies, respectively. We made sure not to introduce the ZAM copies located in germline piRNA clusters of the X chromosome of the RevI-H2i2 line that are involved in the production of ZAM -regulating piRNAs in the germline. smRNA FISH revealed that ZAM RNAs were strongly expressed when these ZAM copies were added to the genome of the flamΔZAM line (Fig. 4d – panels 2 and 3). We also observed a strong invasion of oocytes with chromosome II, where approximately 70% of stage 10 follicles presented ZAM RNAs in the ooplasm, and moderate invasion with chromosome III. Similarly, we observed strong invasion of the oocyte when we added three euchromatic ZAM copies located on the telomere side of the X chromosome of the RevI-H2 line to the flamΔZAM genome (Fig. 4d – panel 4). Overall, our findings show that in the absence of ZAM -derived piRNAs in the somatic follicle cells and in the germline, transcripts from functional ZAM copies massively invade the oocytes. Additionally, our results demonstrate that the presence of a solo-LTR of ZAM (454 bp) in the flam piRNA cluster of the flamΔZAM line was not sufficient to silence ZAM expression in follicle cells (Supplementary Figure 4a ). The three ZAM copies added to the X chromosome of the flamΔZAM line consist of one full length ZAM insertion (ZAM-fl), one ZAM-v2 and one ZAM-v3. Utilizing the sequence specificity of each insertion, we conducted RT-PCR analysis to determine which copies were expressed. The results revealed that ZAM-fl, ZAM-v2 and ZAM-v3 copies are expressed in RevI-H2i2 ovaries as well as when joined to the flamΔZAM genome (Supplementary Figure 4b ). An important observation was that the flamΔZAM flies that contain the three functional ZAM copies on the X chromosome displayed atrophied ovaries and reduced fertility compared with the control flamΔZAM flies that lack functional ZAM copies (Fig. 4e, f ). Specifically, 90% of flamΔZAM females with active ZAM copies did not lay eggs. These data indicate that the reactivation of one single errantivirus in a patch of follicle cells can induce severe fertility defects. These results suggest that when ZAM piRNAs are produced in the germline, they contribute to ensure not only genome integrity but also fertility by protecting the oocytes against ZAM invasion. No initial small RNA response takes place after ZAM reactivation The reactivation of an errantivirus, such as ZAM , in a genetic context where the piRNA pathway is functional provides a unique opportunity to examine the genomic immune response to TE reactivation and germline invasion. piRNAs and siRNAs are the two main classes of small RNAs produced to control the expression of transposable elements and counteract viral infection, respectively. Moreover, invading viral RNAs can be processed to small RNAs to initiate a primary response [40] , [41] . To characterize the small RNA response upon ZAM reactivation, we sequenced small RNAs that are complexed with Argonaute proteins (named here regulatory piRNAs) from flamΔZAM ovaries containing two or four potentially functional ZAM copies. In the flamΔZAM line, there were no de novo ZAM piRNAs (23 to 29 nt) produced upon ZAM reactivation, despite germline invasion. Indeed, only few sense and antisense ZAM piRNAs were detected in the ovaries of the flamΔZAM line that contained functional ZAM copies (Fig. 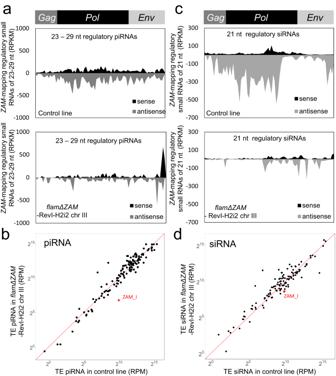Fig. 5: No initial piRNA and siRNA response afterZAMretrotransposon reactivation. aDensity plot of regulatory piRNAs along theZAMinternal sequence in ovaries from a control line (white-sKD) and from theflamΔZAM-RevI-H2i2 chr III line (up to 3 mismatches).bScatter plots showing the normalized counts of regulatory piRNAs mapping to individual internal TE sequences in control ovaries (white-sKD) versusflamΔZAM-RevI-H2i2 chr III ovaries. piRNA counts, mapped allowing up to 3 mismatches, were normalized per million of genome-mapping piRNAs (RPM, here in logarithmic scale).cDensity plot ofZAM-mapping regulatory siRNAs (21nt small-RNAs complexed with Argonaute proteins) along theZAMinternal sequence produced in control (white-sKD) and inflamΔZAMRevI-H2i2 chr III ovaries (0-1 mismatch).dScatter plot showing the normalized counts of antisense regulatory siRNAs mapping to individual internal TE sequences in control ovaries (white-sKD) versusflamΔZAMRevI-H2i2 chr III ovaries. Antisense siRNA counts, mapped allowing up to 1 mismatch, were normalized per million of genome-mapping siRNAs (RPM, here in logarithmic scale). 5a , Supplementary Figure 5a ). Moreover, this lack of piRNA production concerned only ZAM . The level of regulatory piRNAs targeting other TEs was not reduced (Fig. 5b , Supplementary Figure 5b ). Fig. 5: No initial piRNA and siRNA response after ZAM retrotransposon reactivation. a Density plot of regulatory piRNAs along the ZAM internal sequence in ovaries from a control line ( white -sKD) and from the flamΔZAM -RevI-H2i2 chr III line (up to 3 mismatches). b Scatter plots showing the normalized counts of regulatory piRNAs mapping to individual internal TE sequences in control ovaries ( white-sKD ) versus flamΔZAM -RevI-H2i2 chr III ovaries. piRNA counts, mapped allowing up to 3 mismatches, were normalized per million of genome-mapping piRNAs (RPM, here in logarithmic scale). c Density plot of ZAM -mapping regulatory siRNAs (21nt small-RNAs complexed with Argonaute proteins) along the ZAM internal sequence produced in control ( white -sKD) and in flamΔZAM RevI-H2i2 chr III ovaries (0-1 mismatch). d Scatter plot showing the normalized counts of antisense regulatory siRNAs mapping to individual internal TE sequences in control ovaries ( white-sKD ) versus flam Δ ZAM RevI-H2i2 chr III ovaries. Antisense siRNA counts, mapped allowing up to 1 mismatch, were normalized per million of genome-mapping siRNAs (RPM, here in logarithmic scale). Full size image We sequenced total small RNAs in vret- or yb -sKD ovaries where ZAM was also reactivated. Surprisingly we observed sense ZAM -mapping small RNAs of various sizes, including 23-29 nt small RNAs that are not produced in a white -sKD control condition (Supplementary Figure 5c ). However, the sense 23-29 nt ZAM -derived small RNAs detected in yb - and vret -sKD ovaries did not display uridine bias at the 5’ end, a feature of mature primary piRNAs (Supplementary Figure 5d ). Furthermore, these sense ZAM -mapping small RNAs were not immunoprecipitated with Piwi proteins. We detected almost no Piwi-bound sense or antisense ZAM -mapping piRNAs in vret- or yb- sKD ovaries (Supplementary Figure 5e ). In addition, no sense regulatory ZAM piRNAs complexed with Argonaute proteins were detected in vret- sKD ovaries (Supplementary Figure 2f ). These results suggest that the sense ZAM -mapping small RNAs are most likely degradation products of excess ZAM sense transcripts and not piRNAs. Thus, in these different conditions, we did not detect any primary piRNA response either in the somatic cells where ZAM is expressed or in the oocyte that it invades. Given that the ZAM errantivirus shares some structural and functional characteristics with retroviruses, we also asked whether ZAM reactivation could trigger a siRNA response. For this, we analyzed the production of 21 nt small RNAs complexed with Argonaute proteins (regulatory siRNAs). Similar levels of ZAM 21 nt small RNAs were produced in a control line and in the flamΔZAM line with functional ZAM copies (Fig. 5c ). Globally, the production of 21 nt small RNAs in this line was comparable to the control for all TEs, including ZAM (Fig. 5d ). ZAM -mapping 21 nt small RNAs were slightly increased only in the vret -sKD condition, compared to the white -sKD control line without ZAM expression (Supplementary Figure 5f ). Overall, our results suggest that no or very few siRNAs that could protect ovaries from ZAM activity are produced upon activation of this errantivirus in follicle cells. Therefore, we propose that no innate small RNA response is triggered in the lines where ZAM is reactivated, suggesting that ZAM will not be brought under control until the establishment of specific adaptive immunity and immune memory. The discovery that piRNAs produced in germ cells not only restrict TE expression in the germline itself but also counteract the invasion of errantiviruses from adjacent cells reveals a novel role of piRNAs produced locally as an effective defense mechanism at the tissue scale. When piRNAs against ZAM are produced in the germline, ZAM transcripts are limited to a patch of follicle cells and flies are fertile. Conversely, in the absence of ZAM -derived piRNAs in the germline, transcripts from functional ZAM copies massively invade the oocytes and are even transmitted to the embryos. At the molecular level, our study revealed that piRNAs produced in nurse cells and dumped into the oocyte can target RNAs produced by follicle cells and delivered to the oocyte. It is tempting to speculate that the ZAM RNAs arriving from somatic cells are targeted by complementary antisense piRNAs and degraded through the ping-pong cycle (reviewed in [33] ). This would result in the production of ZAM sense piRNAs, thus participating in the amplification of the pool of piRNAs against ZAM and strengthening the defense mechanism against the invasion. Transposition in the germ cell genome is crucial for TE propagation in a population because it allows the vertical transmission of new insertions. At the time of invasion (e.g. in the flam∆ZAM line), no ZAM -derived piRNA was produced in somatic or germ cells. Therefore, this condition could be compared to what happens when a TE first enters a new species by horizontal transfer. In this case, according to several studies, an initial transposition burst occurs that leads to TE accumulation in the genome before the induction of an adaptive response by the host to control transposition [42] , [43] , [44] , [45] , [46] , [47] . We found at least 17 new ZAM insertions in the RevI-H2i2 genome, testifying that ZAM actively transposed. Surprisingly, we identified three ZAM insertions in the same germline piRNA cluster on the X chromosome. It has been proposed that two different mechanisms can explain the de novo piRNA production required to specifically silence a novel invading TE. Indeed, piRNAs can be produced from a new TE insertion into a pre-existing piRNA cluster, and also by stand-alone TE insertions converted into piRNA-producing loci [48] , [49] , [50] , [51] . Interestingly, when active ZAM copies are added into a flamΔZAM genetic background, these copies do not produce regulatory ZAM -derived piRNAs and are not converted into piRNA producing regions. Actually, ZAM should be transcriptionally inactive in the germline because ZAM expression is regulated by the somatic transcription factor Pointed [34] . Therefore, although the contribution of individual copies needs to be investigated, our data strongly suggest that germline ZAM piRNAs originate at least in part from piRNA clusters. In line with our findings, computer simulations of the TE invasion dynamics suggested that several insertions in piRNA clusters are likely to be required to stop the invasion in the germline [52] . Conversely, we found that a single insertion in a somatic piRNA cluster, such as flamenco , is sufficient for TE silencing in the somatic follicle cells, as previously suggested [25] . Indeed, we show here that in follicle cells, the flamenco piRNA cluster acts alone as the principal regulator of transposon activity. A precise deletion of the internal part of the ZAM TE inserted in flamenco leads to complete derepression of functional ZAM copies. Surprisingly, it seems that reactivation of this errantivirus in only a patch of somatic cells can lead to severe fertility defects. However, in the germline, the deletion of the three most highly expressed germline piRNA clusters (42AB, 38 C, and 20 A) affected neither fertility nor TE silencing [50] . This could be explained by the fact that in the germline, but not in somatic cells, redundancy in piRNA production among different piRNA clusters is observed, with probably multiple piRNA clusters involved in the silencing of the same TE. Moreover, many TE copies have acquired mutations and are non-functional for transcription or for transposition. In the flam∆ZAM line, although no ZAM piRNA was produced, we did not detect any ZAM expression. However, when we introduced functional copies of ZAM , ZAM was expressed demonstrating that depending on the genetic background, the transposon landscape varies and functional copies can be absent or present. In general, the TE content varies considerably among populations [49] , [53] . Interestingly, we identified ZAM copies with a deletion that affects the pol gene. The copy numbers of this ZAM variant ZAM-v2 and of ZAM full-length elements (ZAM-fl) that have transposed in the RevI-H2 line are similar (4 and 6 copies respectively), suggesting that even this ZAM variant can transpose very efficiently. Studies in different organisms have shown that TEs rapidly diversify. For instance, the mariner DNA transposon is present in 68 different versions in grass genomes [54] . Such rapid diversification certainly promotes speciation of new families of active TEs. One interesting question is how ZAM RNAs transit into the oocyte and at which stage during Drosophila oogenesis ZAM transposes in germ cells. We noticed that ZAM RNAs, although transcribed in follicle cells, were deposited and accumulated at the posterior pole of early embryos, where future germ cells cellularize. ZAM might have evolved to preferentially mobilize in the dividing primordial germ cells of the offspring instead of the developing oocyte, which is not in a phase favorable to transposition because of its prolonged arrest in prophase I associated with highly compacted chromatin [55] . Previous experiments demonstrated that ZAM RNAs accumulate in follicle cells when vitellogenesis is defective, suggesting that ZAM transmission to the oocytes requires functional vitellogenin trafficking [11] (Supplementary Movie 1 ). Moreover, errantiviruses, such as ZAM and Gypsy , can form pseudo-viral particles in follicle cells when they are expressed [8] , [10] , [11] , [15] . ZAM Gag and Env proteins are expressed in RevI-H2i2 follicle cells. Retroviral envelope glycoproteins undergo proteolytic processing by cellular serine endoproteases (furin and proprotein convertases), in order to produce the two functional subunits, a glycosylated hydrophilic polypeptide (SU) and a transmembrane domain (TM). This step is necessary to achieve protein competence to promote membrane fusion and virus infectivity [56] , [57] . The errantiviral env gene, acquired from insect baculovirus [2] , encodes a protein whose function is analogous to that of retroviral Env protein, which is responsible for infectious properties. Indeed, ZAM Env protein is composed of an SU, a TM and an Arg–X–Lys–Arg conserved domain, which is considered to be a furin consensus proteolytic cleavage site [28] , [57] , [58] . A recent study demonstrated that intracellular retrotransposition of the Gypsy errantivirus can occur in the absence of the Env protein, while intercellular transmission requires a functional Env [10] . Currently, whether ZAM can transpose intracellularly, in follicle cells, and the exact mechanisms (Env protein dependent or independent) used for ZAM transmission to the oocyte are unknown. Once a virus enters the target cells, several scenarios for retrovirus uncoating have been proposed. Recent advances on the HIV-1 strongly suggest an uncoating at the nuclear pore and within the nuclear compartment [59] . Errantiviruses also encode Gag proteins which are capable of mediating the assembly of virus-like particles. However, there are significant differences between these proteins and retroviral Gag proteins, which might lead to a different uncoating process for errantiviruses [60] . In our study, we observed the loss of ZAM RNA in the oocyte when germline ZAM -derived piRNAs are produced. We can hypothesize that the ZAM capsid is dissociated soon after entry into the oocyte and that piRNAs can therefore easily target ZAM RNAs. It is also possible that ZAM RNAs are still encapsidated in the oocyte, but the capsid does not protect the ZAM RNA from piRNAs and their associated endonuclease. Previous studies on virus-like particles of the yeast Ty retrotransposon suggest that these particles form open structures that leave the RNA at the interior of the capsid accessible to RNase [61] , [62] . It has been proposed that in different species, an “innate” response at the piRNA or siRNA level can be initiated in the gonads upon retrovirus invasion ( [41] , [63] , [64] , [65] , [66] , [67] , [68] ). We found that no clear innate small RNA response is triggered upon ZAM reactivation in Drosophila ovaries. Total small-RNA sequencing after ZAM reactivation revealed the presence of sense ZAM -mapping small RNAs, but they lack characteristics of siRNAs or piRNAs. We hypothesize that these sense small RNAs are degradation products generated when there is an excessive amount of ZAM RNAs. Altogether, these results show that no initial small RNA response is mounted upon ZAM reactivation, leaving follicle cells, where ZAM is expressed, and also oocytes unprotected against ZAM transposition. Our findings suggest that the piRNA response is a robust response that, in the case of ZAM , must be established either in the follicle cells or in the germ cells to efficiently control the invading TE. However, the time required for developing a robust piRNA response to sustainably control TE transposition remains unknown. Lastly, it is thought that the piRNA pathway has no antiviral role in Drosophila [69] . However, it would be interesting to determine whether this is also true if parts of the viral genome are integrated into a germline piRNA cluster during infection. Fly stocks, transgenic lines, and crosses Flies were maintained at 25 °C under a light/dark cycle and 60% humidity. Between 3 and 6 days after hatching, flies were used for experiments. The RNAi lines against components of the piRNA pathway used in this study are listed in Supplementary Data 2 . Isogenic lines from the RevI-H2 stock were generated by crossing a single female with a single male for five generations. Germline and somatic knock-down have been performed using the nanos-gal4 and the traffic-jam-gal4 driver lines respectively (Supplementary Data 2 ). The Drosophila line carrying the ZAM sensor is described in [30] . The sensor expresses the GFP reporter gene under the control of an inducible Upstream Activation Sequence promoter (UASp) and harbors a ZAM fragment in its 3′-UTR (pGFP- ZAM ). Single-molecule RNA fluorescence in situ hybridization (smRNA FISH) in ovaries and embryos All reagents are described in Supplementary Data 7 . ZAM smRNA FISH was performed using 48 probes that target ZAM transcripts in a region that is absent in the ZAM inserted in the flamenco piRNA cluster to detect only transcripts of active ZAM copies (sequences in Supplementary Data 3 ). Ovaries from 3 to 6-day-old flies were dissected in Schneider’s Drosophila Medium and fixed in Fixing Buffer (4% formaldehyde, 0.3% Triton X-100, 1x PBS) for 20 min at room temperature, rinsed three times in 0.3% Triton X-100, once in PBS, and permeabilized in 70% ethanol at 4 °C overnight. Permeabilized ovaries were rehydrated in smRNA FISH wash buffer (10% formamide in 2x SSC) for 10 min. Ovaries were resuspended in 50 µL hybridization buffer (10% dextran sulfate, 10% formamide in 2x SSC) supplemented with 1 µL of smRNA FISH probes. Hybridization was performed with rotation at 37 °C overnight. Ovaries were then washed twice with smRNA FISH wash buffer at 37 °C for 30 min and twice with 2xSSC solution. Then, DNA was stained with DAPI (1/500 dilution in 2x SSC) at room temperature for 20 min. Ovaries were mounted in 30 µL Vectashield mounting medium and imaged on a Zeiss LSM-980 or Zeiss LSM-800 confocal microscope. The resulting images were processed using FIJI/ImageJ. The RNA signal specificity was confirmed by adding 1 mg/mL of RNase A in 2x SSC for 2 h before the hybridization step. For embryo staining, flies were caged and fed yeast paste. Embryos (0–2 h) were collected, dechorionated in 50% bleach for 4 min and rinsed in water. Eggs were fixed in 4% paraformaldehyde/heptane for 20 min, devitellinized by vigorous shaking in 100% methanol and stored in methanol at −20 °C. Embryos were rehydrated with 1:1 methanol in 1xPBS, 0.1% Tween-20 for 5 min and twice in 1xPBS, 0.1% Tween-20. Embryos were resuspended in smRNA FISH wash buffer (10% formamide in 2x SSC) for 10 min and then processed for smRNA FISH as described for ovaries. Immunostaining combined with smRNA FISH was performed by adding primary antibodies to the smRNA FISH probes in the hybridization buffer and incubating at 37 °C overnight. Embryos were washed twice with smRNA FISH wash buffer and incubated with the secondary antibody for 90 min. After two washes in 2x SSC, embryos were mounted in 30 µL Vectashield mounting medium. Immunofluorescence analysis of ovaries and embryos All reagents are described in Supplementary Data 7 . Ovaries from 3–6-day-old flies were dissected in supplemented Schneider’s medium, ovarioles were separated, and the muscle sheath was removed before fixation to obtain undistorted follicles. Then, ovaries were fixed in 4% formaldehyde/1x PBS/2% Tween-20 for 15 min, rinsed three times with 1x PBS/2% Tween-20, and incubated 2 hours in PBT (1x PBS, 0.1% Triton X-100, 1% BSA). Ovaries were incubated with primary antibodies in PBT at 4 °C overnight (antibodies are described in Supplementary Data 4 ). After three washes in PBT, ovaries were incubated with the corresponding secondary antibodies coupled to Alexa-488 or Cy3 for 90 min. After two washes in 1x PBS, DNA was stained with DAPI (1/500 dilution in 1x PBS) for 20 min. Ovaries were mounted in 30 µL Vectashield mounting medium and imaged on a Zeiss LSM-980 or Zeiss LSM-800 confocal microscope. The resulting images were processed using FIJI/ImageJ. RT-qPCR analysis of transposon expression All reagents are described in Supplementary Data 7 . 10-20 pairs of dissected ovaries were homogenized in TRIzol reagent. Following DNase I treatment, cDNA was prepared from 1 µg RNA by random priming of total RNA using Superscript IV Reverse Transcriptase. Quantitative PCR was performed with Roche FastStart SYBR Green Master on a the Lightcycler® 480 Instrument. RT-qPCR was used for quantification of transposon mRNA levels (primer sequences in Supplementary Data 5 ). All experiments were done with three biological replicates and with technical triplicates. Steady-state RNA levels were calculated from the threshold cycle for amplification with the 2 −∆∆CT method; rp49 was used for normalization. Immunoprecipitation of Piwi-ribonucleoprotein complexes All reagents are described in Supplementary Data 7 . For each genotype, 50 pairs of ovaries from 3-6-day-old flies were dissected, lysed in 1 ml lysis buffer (20 mM HEPES-NaOH at pH 7.0, 150 mM NaCl, 2.5 mM MgCl 2 , 250 mM sucrose, 0.05% NP40, 0.5% Triton X-100, 1x Roche-Complete). Samples were cleared by centrifugation at 10,000× g at 4 °C for 10 min. Extracts were incubated with rotation with rabbit polyclonal anti-Piwi antibodies (4 µg per sample) at 4 °C for 4 h followed by overnight incubation with Dynabeads TM Protein A (50 µl, Invitrogen, 10002D) at 4 °C with rotation. Before incubation, beads were equilibrated in NT2 buffer (50 mM Tris-HCl, pH 7.4, 150 mM NaCl, 1 mM MgCl 2 , 0.05% NP40). Beads were washed twice with ice-cold NT2 and twice with NT2 in which NaCl concentration was adjusted to 300 mM. Nucleic acids that co-immunoprecipitated with Piwi were isolated by treating beads with 0.7 mg/ml proteinase K in 0.3 ml proteinase K buffer (0.5% SDS, 10 mM Tris-HCl pH 7.4, 50 mM NaCl, 5 mM EDTA), followed by phenol/chloroform extraction (phenol at neutral pH) and ethanol precipitation. DNA Isolation, Oxford Nanopore Technology sequencing and genome analysis All reagents are described in Supplementary Data 7 . DNA was extracted from 200 RevI-H2i2 females using the Qiagen Blood & Cell Culture DNA Midi kit. The genomic DNA quality and quantity were evaluated using a Femto Pulse (Agilent) and a Qbit 3.0 (Invitrogen) respectively. Oxford Nanopore Technology (ONT) sequencing was performed by I2BC (Gif-sur-Yvette, France) using five micrograms of genomic DNA. Adapter-trimmed ONT reads were analyzed using NCBI Blastn ( https://blast.ncbi.nlm.nih.gov/Blast.cgi ) or command-line Blastn (Blastn 2.8.1). The RevI-H2i2 ONT reads containing ZAM insertions were detected by Blastn with the reference ZAM [22] , Repbase ZAM_I and ZAM_LTR sequences ( https://www.girinst.org/repbase/ [31] ,). The ZAM containing reads were then recovered with bedtools getfasta ( https://bedtools.readthedocs.io/en/latest/content/tools/getfasta.html [70] ,). The ZAM insertion sites where determined using Blastn of the ZAM containing reads to the D. melanogaster Release 6 genome ( http://flybase.org ). The absence of empty sites, without a given ZAM insertion, was verified by Blastn of the respective empty insertion sites, recovered from the D. melanogaster Release 6 genome, to all ONT reads. Sequencing data are available in NCBI GEO database, accession GSE213456 . RNA-sequencing and analysis 3 independent total RNA extractions from 30 ovaries from 3-6-day-old RevI-H2i2 flies using Trizol (Invitrogen) were performed. Strand-specific libraries for RNA sequencing (RNA-Seq) were constructed at BGI. 1 µg of total RNA was used to prepare mRNA library using MGIEasy RNA Library Prep kit and sequenced as PE150 reads on the DNBSEQ G400 sequencer, and adapter-clipped reads were provided by BGI. The data were analyzed on the local Galaxy platform using HISAT2 alignment (Galaxy Version 2.1.0). The reads were first mapped to ZAM-fl and to ZAM-v2 using the “Disable spliced alignment” option. The mapped reads were then aligned to ZAM_I sequence (Repbase) with the default options, i.e. allowing split alignment. Reads were visualized using “Integrative Genomics Viewer” version 2.16.1. The coverage of RNA-seq reads corresponding to ZAM-v2 was determined as the number of split reads specific to the ZAM-v2 deletion at positions ZAM_I:5494-6120, normalized to the average coverage of the pointed transcript. Coverage of RNA-seq reads corresponding to ZAM-fl and ZAM-v2 was determined as the number of nonsplit reads at position 5495, the left edge of the deletion, normalized to the average coverage of the pointed transcript. Only the left edge was used for this purpose, as the right edge of the deletion is also mapped by reads corresponding to ZAM variants with other internal deletions (green in Fig. 1a ). RNA sequencing data are available in NCBI GEO database, accession GSE235966 . Small RNA sequencing Regulatory small RNA extraction was performed as described in [71] . Briefly, 50 pairs of ovaries from 3-6-day-old flies were lysed and Argonaute-small RNA complexes were isolated using TraPR ion exchange spin columns (Lexogen, Catalog Nr.128.08). Total RNA also was extracted for some samples (80-100 ovaries for each sample) using the classical TRIzol extraction, followed by 2 S rRNA depletion and size selection before sequencing. Sequencing was performed by Fasteris SA (Geneva, Switzerland) on an Illumina NextSeq550 instrument (13–15 million reads per sample). Illumina small RNA sequencing reads were loaded on the small RNA analysis pipeline sRNAPipe [72] for mapping to the various genomic sequence categories of the D. melanogaster genome (Release 6). For the analysis, 23-29nt genome mappers were selected as piRNAs, and 21nt genome mappers were selected as siRNAs. Genome-unique piRNAs were defined as 23–29 reads that mapped uniquely across the reference genome. piRNAs were mapped to TEs allowing up to 3 mismatches, siRNAs allowing up to 1 mismatch, and genome-unique piRNAs to piRNA clusters as defined in [22] allowing no mismatch. The window size was of 91nt for the entire ZAM , 86 nt for ZAM_I and 140nt for the flamenco region at X:21,769,891..21,789,891 to establish the piRNA density profiles. For comparison between samples, all read counts were normalized by the number of piRNA/siRNA reads used as input (genome-mapped piRNAs or siRNAs, genome-unique piRNAs) and represented in RPM [RPM = read-count * 1,000,000 / (total of genome mapping piRNAs)], or RPKM [RPM = read-count * 1,000,000 / (TE Length/1000) / (total of genome mapping piRNAs)] in the case of density profiles. To assess the ping-pong signature, the counts of 1 to 23nt 5’-overlaps were determined, and the percentage of 10nt 5’-overlaps over the total 1-23nt 5’-overlaps was calculated. The Z-score for 10nt 5’overlaps was determined using the percentages of all 1 to 23nt-long 5’overlaps as a background and was considered significant when it was >1.96. Scatter plots were done with RStudio with antisense piRNAs or siRNAs mapping to the respective internal sequence of TEs (allowing 0-3 mismatches for piRNAs and 0-1 mismatch for siRNAs). All small RNA sequencing done for this study is listed in Supplementary Data 6 . Small-RNA sequencing data are available in NCBI GEO database, accession GSE213368 . Sterility tests For the sterility tests, RevI-H2i2 homozygous females were compared to w 1118 females, and homozygous flamΔZAM females that carry three functional ZAM copies from the RevI-H2 X chromosome were compared to flamΔZAM females without these functional ZAM copies in their genome. Sterility tests were performed at 25 °C. Thirty 3-6-day-old virgin females of each genotype were individually mated with three w 1118 males, and eggs were collected for 24 hours. The number of eggs laid by each female was determined. Then, eggs were kept at 25 °C for another 24 hours before determining the egg hatching rate. The experiment was done twice for a total of approximatively 60 replicates for each condition. Generation of the flamΔZAM line using the CRISPR-Cas9 technology The ZAM copy in the flamenco piRNA cluster was deleted using a pCFD6 plasmid that expresses two single guide RNAs (sgRNAs) under the Gal4/UAS system. The sgRNAs were designed to target genome-unique sequences located upstream and downstream of the flamenco ZAM copy: TTGTAGCGCTCTTCTTCTCT (sgRNA flamΔZAM_1 ) and AGCGCAACCACGTACAGCGA (sgRNA flamΔZAM_2 ). The pCFD6 plasmid harboring these sgRNAs was injected by the Bestgene company into embryos from the BL#9736 stock (Bloomington stock center) for integration of the plasmid into the genomic site 53B2. The obtained flies were crossed with nanos-gal4; UAS-Cas9 flies (BL#54593, Bloomington stock center). Prior to crossing, the X chromosome of each of these lines was replaced by the X chromosome of the Iso1A Drosophila line. After the crosses, 500 lines were derived and screened by PCR using primers specific for the flamenco ZAM copy. The detailed crossing schemes are available upon request. Lines without amplification of internal flamenco ZAM sequences were selected for PCR amplification of the target locus with primers that framed the flamenco ZAM copy and the target sequences of the sgRNAs. The obtained amplicons were sequenced. Reporting summary Further information on research design is available in the Nature Portfolio Reporting Summary linked to this article.